Convergence and coevolution of Hepatitis B virus drug resistance Treatment with lamivudine of patients infected with hepatitis B virus (HBV) results in a high rate of drug resistance, which is primarily associated with the rtM204I/V substitution in the HBV reverse transcriptase domain. Here we show that the rtM204I/V substitution, although essential, is insufficient for establishing resistance against lamivudine. The analysis of 639 HBV whole-genome sequences obtained from 11 patients shows that rtM204I/V is independently acquired by more than one intra-host HBV variant, indicating the convergent nature of lamivudine resistance. The differential capacity of HBV variants to develop drug resistance suggests that fitness effects of drug-resistance mutations depend on the genetic structure of the HBV genome. An analysis of Bayesian networks that connect rtM204I/V to many sites of HBV proteins confirms that lamivudine resistance is a complex trait encoded by the entire HBV genome rather than by a single mutation. These findings have implications for public health and offer a more general framework for understanding drug resistance. Hepatitis B virus (HBV) causes chronic infection in >350 million people worldwide. Cirrhosis, liver failure and hepatocellular carcinoma associated with chronic HBV infections account for ~1 million deaths annually [1] . The HBV genome consists of partially double-stranded DNA of ~3,200 base pairs that replicates via reverse transcription of the pregenomic RNA [2] . Treatment of chronically infected patients with nucleos(t)ide analogues to inhibit the HBV reverse transcriptase (RT) suppresses HBV replication and reduces the risk of liver disease progression. Long-term treatment with RT inhibitors, however, leads to the development of drug resistance [3] , [4] . Lamivudine is one of five RT inhibitors approved for treatment of patients with chronic hepatitis B, and widely used across the world. Lamivudine therapy leads to the appearance of drug-resistant HBV variants in 14–32% of patients during the first year of treatment and ~70% of patients after 5 years [3] . Lamivudine resistance is primarily associated with rtM204I or rtM204V substitution (rtM204I/V) in the YMDD motif of the RT domain. Other mutations that have been reported to be associated with lamivudine resistance include rtA181V/T and several secondary RT mutations, for example, rtV173L and rtL180M [3] . It is estimated that a high rate of mutations in the HBV genome readily results in emergence of all single mutations during chronic HBV infection [5] . Thus, drug-resistance mutations might be present in infected patients even without selective pressure from antiviral drugs. However, the ubiquity of drug-resistance mutations does not completely explain variation in the rate and type of drug resistance in patients receiving antiviral therapy. Besides the size of the viral population, which significantly affects the presentation of specific mutations, epistatic connectivity among HBV genomic sites can have a very important role in establishing the drug-resistance phenotype [6] . Genetic analysis of resistance to nucleos(t)ide inhibitors is usually focused on the RT domain and only infrequently takes into consideration the whole genome of intra-host HBV variants [6] , [7] , [8] . This limits evaluation of epistatic connectivity across the viral genome and its association to drug resistance. In this study, we analysed a large set of whole-genome sequences of the intra-host HBV variants recovered from 11 HBV-infected patients, who were undergoing lamivudine treatment, and showed the important contribution of convergence and site coevolution in lamivudine resistance. 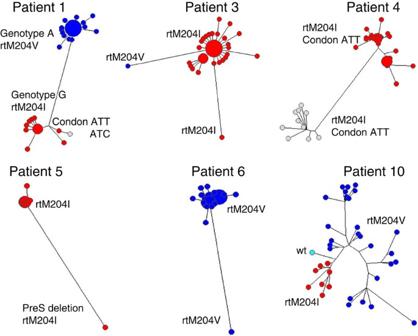Figure 1: Maximum likelihood trees of intra-host HBV variants sampled from patients after lamivudine treatment. The node size is proportional to frequency of the corresponding variant in the viral population. Colours correspond to the codon states at position rt204: rtM204I coded by ATT or ATC is shown in red or grey, respectively; rtM204V is shown in blue (codon GTG); the wild type is shown in cyan (codon ATG). The distance between the two genotype clusters of Patient 1 was plotted 20 times shorter to allow the visualization of minor variants. Intra-host population of lamivudine-resistant HBV variants HBV whole-genome quasispecies were sampled from 11 patients who experienced virological breakthrough during lamivudine treatment ( Table 1 ). A total of 395 whole-HBV genomes were sequenced using end-point limiting-dilution RT–polymerase chain reaction (PCR) [9] . On an average, 36 HBV genomes were sampled from each patient. Patients were infected with HBV genotypes A ( n =4), B ( n =1), C ( n =2) and D ( n =2). Patient 1 was infected with mixed genotypes A and G, and Patient 9 with a recombinant genotype A/G strain ( Table 1 ). The rtM204I/V substitution was detected in all patients except Patient 9. This patient did not have any known lamivudine-resistance-associated mutations. Table 1 Virological characteristics and YMDD patterns of patients on lamivudine treatment. Full size table Analysis of mutations in the YMDD motif showed that intra-host HBV populations may have more than one type of lamivudine-resistance mutations. For example, the HBV genotype A variants in Patient 1 contained the rtM204V substitution, whereas variants of genotype G in the same patient contained rtM204I ( Fig. 1 ). Codon usage additionally contributed to the genetic heterogeneity underlying lamivudine-resistance. For example, ATC coding for isoleucine in YIDD was found in one genome among the ten genotype G variants in Patient 1, while all other variants contained ATT. Patient 4 was infected with two HBV genotype B subpopulations ( Fig. 1 ), both containing the rtM204I substitution. However, in one subpopulation the isoleucine was encoded by ATC, whereas in the other subpopulation it was encoded by ATT. Nine of ten HBV variants containing ATC ( Fig. 1 ) harboured additional substitution rtA181T that also confers decreased susceptibility to lamivudine and adefovir [10] . In Patient 10, 23% of all variants contained the rtM204I substitution, whereas the remainder contained rtM204V. Among 44 HBV variants identified in Patient 3, 43 contained rtM204I, while 1 variant contained rtM204V. This variant was different from the major cluster at a minimum of six positions. It was one of two most genetically distinct variants ( Fig. 1 ) and thus, represents a minority HBV subpopulation. Figure 1: Maximum likelihood trees of intra-host HBV variants sampled from patients after lamivudine treatment. The node size is proportional to frequency of the corresponding variant in the viral population. Colours correspond to the codon states at position rt204: rtM204I coded by ATT or ATC is shown in red or grey, respectively; rtM204V is shown in blue (codon GTG); the wild type is shown in cyan (codon ATG). The distance between the two genotype clusters of Patient 1 was plotted 20 times shorter to allow the visualization of minor variants. Full size image All the HBV variants in Patients 5 and 6 contained rtM204I or rtM204V, respectively. However, in Patient 5, one variant differed from all other variants at eight positions and contained two deletions of 30 and 57 bp in the preS1 region ( Fig. 1 ). In Patient 6, a single variant was found to be different from the main HBV cluster at 24 positions, with one substitution that additionally changed YVDD to YVND ( Fig. 1 ). Patient 9, who developed drug resistance through a YMDD-unrelated mechanism, also contained one HBV-outlier variant, which differed from the main intra-host HBV population at 19 positions. Thus, Patients 5, 6 and 9 were infected with complex lamivudine-resistant HBV populations that contained distinct minority variants. Collectively, the aforementioned observations indicate that lamivudine resistance was independently acquired by more than one HBV variant in each patient studied, and point to the frequent availability of the lamivudine-resistance mutations and homoplastic nature of the resistance in intra-host HBV populations. Lamivudine-induced changes in intra-host HBV populations To analyse adaptation of intra-host HBV populations to lamivudine treatment, whole-genome sequences of intra-host HBV variants from pre-treatment samples ( n =244) were additionally analysed in Patients 6–11. Comparison of the variants showed considerable changes in the genetic structure of intra-host HBV populations during treatment ( Fig. 2 ). HBV populations identified before and after treatment were distinctly different in all patients. In Patients 6 and 9, the rtM204I substitution was identified in a single clone of pre-treatment HBV populations but these clones were not present in their post-treatment populations ( Table 1 ). 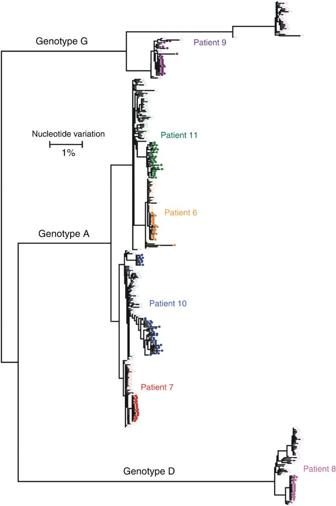Figure 2: Maximum likelihood trees of intra-host HBV variants from six patients. HBV populations sampled from patients infected with genotypes A (n=4), D (n=1), G (n=1) before (open circles) and after (colour-filled circles) lamivudine treatment. Each colour presents a single patient. Figure 2: Maximum likelihood trees of intra-host HBV variants from six patients. HBV populations sampled from patients infected with genotypes A ( n =4), D ( n =1), G ( n =1) before (open circles) and after (colour-filled circles) lamivudine treatment. Each colour presents a single patient. Full size image The pre-treatment HBV variants in Patients 8 and 9 were organized into two major subpopulations. Interestingly, their HBV genetic diversity was greatly reduced after treatment, when only a single subpopulation successfully established lamivudine resistance ( Fig. 2 ). The subpopulation, which was not found after treatment in Patient 8, contained a large deletion of 183 bp in the preS region at positions 2,984–3,166. Although Patient 9 was infected with genotype G and recombinant genotype A/G variants, no constituents of the genotype G subpopulation were identified after treatment. The finding is surprising because the genotype G subpopulation contained a variant manifesting rtM204I. These observations in the two patients indicate significant differences in the capacity to evolve toward lamivudine resistance among the intra-host HBV variants. In Patient 7, the HBV genetic diversity, as measured by Shannon entropy (Sn), was also significantly reduced after treatment (6.3×10 −4 versus 3.6×10 −4 ; paired samples t -test, P =0.0085). The HBV genetic diversity was not significantly different in Patient 6 (paired samples t -test, P =0.7104) and Patient 11 (paired samples t -test, P =0.0849). The HBV genetic diversity was significantly increased after treatment only in Patient 10 (1.1×10 −3 versus 2.3×10 −3 ; paired samples t -test; P <0.0001). The frequency distribution of HBV variants was similar in Patients 6, 7, 10 and 11 before and after therapy ( Fig. 3 ). HBV populations in Patients 6 and 7 contained high-frequency variants, with only ~47–80% of all sampled HBV sequences being unique. The star-like phylogeny of HBV populations in these two patients after treatment ( Fig. 3 ) is consistent with derivation of these populations from a single lamivudine-resistant HBV variant. However, the complexity of the populations did not significantly change following treatment, so whether lamivudine-resistant populations originated from a single variant is uncertain. By contrast, 93–100% of HBV variants in Patients 10 and 11 were unique; suggesting that adaptation to lamivudine was not associated with strong bottleneck events. 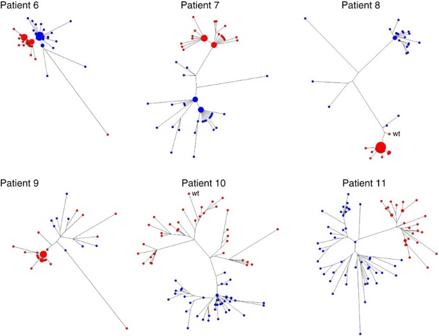Figure 3: Maximum likelihood trees of intra-host HBV variants sampled before and after lamivudine therapy. HBV variants were sampled from Patients 6–11 before (blue) and after (red) treatment with lamivudine. The node size is proportional to frequency of the corresponding variant in the viral population. For Patients 8 and 9, only pre-treatment subpopulations that were genetically closest to the resistant variants are shown. Figure 3: Maximum likelihood trees of intra-host HBV variants sampled before and after lamivudine therapy. HBV variants were sampled from Patients 6–11 before (blue) and after (red) treatment with lamivudine. The node size is proportional to frequency of the corresponding variant in the viral population. For Patients 8 and 9, only pre-treatment subpopulations that were genetically closest to the resistant variants are shown. Full size image We identified a total of 81 sites in the HBV genome that showed significant changes (analysis of molecular variance (AMOVA), P <0.05) in nucleotide frequencies between pre- and post-treatment populations of all six patients. In Patients 8 and 9, only subpopulations that persisted post treatment were considered for analysis. HBV populations in Patients 6 and 7 had significant changes at 5 sites, those in Patient 9 at 7 sites, and those in Patients 8, 10 and 11 at 26, 27 and 25 sites, respectively. Exclusion of the corresponding sites from phylogenetic analysis of HBV variants in each patient resulted in complete intermixing of both pre- and post-treatment HBV populations, indicating essential reduction in genetic differences between these populations. The genetic distance between the pre- and post-treatment populations was different among patients, being approximately four to five times greater for Patients 8, 10 and 11 than for Patients 6, 7 and 9. Besides the sites for the primary (rtM204V/I) and secondary (rtL180M) lamivudine-resistance mutations identified in five patients, only one additional site with significant changes in intra-host populations was shared by HBV in three patients and four sites by HBV in two patients. All other sites ( n =74) were unique for HBV in each patient, indicating a limited degree of common genetic changes during lamivudine treatment among HBV populations in the six patients. Origin of lamivudine-resistant HBV populations Phylogenetic analysis of HBV populations sampled from Patients 6 to 11 showed that some pre-treatment HBV variants were genetically close to the respective lamivudine-resistant population ( Fig. 3 ), which seems to suggest that these variants served as sources for the resistant population. However, such a conclusion is not warranted for all six patients. Assuming parsimony of evolution toward lamivudine resistance, we calculated the average maximum likelihood (ML) distances among all HBV sequences to assess the origin of the lamivudine-resistant HBV variants. For Patients 8 and 9, the analysis was conducted using only pretreatment subpopulations, which were genetically closest to the resistant HBV variants. 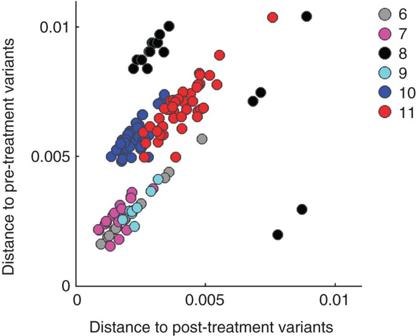Figure 4: Scatterplot of distances among intra-host HBV variants of six patients. Genetic distances are shown for Patients 6–11. Each pre-lamivudine sequence was plotted according to its value in two dimensions: the average distance to all other pre-treatment variants (xaxis) and the average distance to all other post-treatment variants (yaxis). Figure 4 shows a scatter plot of the distances for each patient, where each pre-treatment sequence is plotted according to two variables: first, its average distance to all other pre-treatment sequences( C ), which is a measure of centrality of the sequence in the variant cloud at the time of sampling; and second, its average distance to all post-treatment sequences ( D ), a measure of relatedness of the sequence to the lamivudine-resistant variants. It is important to note that, with the exception of HBV populations in Patients 10 and 11, the most central pretreatment sequences were also the most frequent. A significant positive correlation was found between these two variables for HBV populations in Patients 6, 7, 9, 10 and 11 (Patient 6: r =0.9998, P =1.82E−43; Patient 7: r =0.7034, P =4.26E−05; Patient 9: r =0.8988, P =2.40E−03; Patient 10: r =0.7028, P =2.11E−07; and Patient 11: r =0.8433, P =1.91E−13). This finding indicates that post-treatment HBV populations are genetically close to the most central variants from pre-treatment HBV populations in the five patients. The supposition that lamivudine-resistant HBV populations directly originated from the pre-existing high-centrality variants is to some extent applicable to Patients 6 and 9 only, in whom the main post-treatment HBV populations differed from the pre-treatment variants at a few ( n =2–4) genomic positions (for Patient 9, only recombinant A/G subpopulation was considered.). Figure 4: Scatterplot of distances among intra-host HBV variants of six patients. Genetic distances are shown for Patients 6–11. Each pre-lamivudine sequence was plotted according to its value in two dimensions: the average distance to all other pre-treatment variants ( x axis) and the average distance to all other post-treatment variants ( y axis). Full size image In Patient 6, one major post-treatment HBV variant differed from the major pre-treatment variant by only rtM204V and rtL180M. Nevertheless, close genetic relatedness to sequences with the high C value does not implicate a single source for the resistant HBV variants. Indeed, analysis of phylogenetic trees suggests that the lamivudine-resistant populations in Patients 6 and 9 are polyphyletic ( Fig. 3 ). In Patient 7, HBV populations before and after treatment contained two high-frequency variants. Strikingly, the major variants in each population differed from each other by the same substitution at the same position, rtP1S, and between populations by four substitutions at the same positions, with two of these substitutions being rtM204V and rtL180M. Together with the finding of similarity of the variant-frequency structure of pre- and post-treatment HBV populations, these observations suggest that two major pre-therapy variants gave origin to two major lamivudine-resistant variants, despite the pre-treatment population having contained minority variants that were phylogenetically closer to the post-treatment population ( Fig. 3 ). The post-treatment HBV population in Patient 10 did not contain high-frequency variants. The phylogenetic tree of this population has five major branches. One branch represents a cluster of closely related sequences that contain the rtM204I substitution whereas the other four branches contain rtM204V. One variant of this cluster is wild type, suggesting that it represents the pre-treatment minority HBV subpopulation, which served as a source for subsequent resistant variants containing rtM204I. The complex phylogenetic structure of the post-treatment population constituted of highly diverse variants (Sn=2.3×10 −3 ), the presence of >1 type of lamivudine-resistance substitutions, and the significantly large genetic distance of this population from the pre-treatment population indicate that many lamivudine-resistant variants independently evolved from minority pre-treatment variants. The HBV population in Patient 11 also did not contain high-frequency variants ( Fig. 3 ). This similarity between Patients 10 and 11 suggests the extensive parallel evolution toward lamivudine resistance in Patient 11 as well. Thus, the phylogenetic relationships within the post-treatment HBV population in Patients 10 and 11 reflect phylogenetic relationships among immediate ancestors of the lamivudine-resistant variants rather than a single-source origin of resistance. HBV variants in Patient 8 showed negative correlation between C and D ( Fig. 4 ; r =−0.6062; P =1.69E−03). Inspection of the phylogenetic tree readily shows that one minority pre-treatment subpopulation, which was composed of only 2 variants, was genetically close to the post-treatment population ( Fig. 3 ). The post-treatment variant, which was closest to this subpopulation, was wild type, suggesting that these three variants (two from pre- and one from post-treatment populations) were related to a minority pre-treatment subpopulation that was a source for the lamivudine-resistant HBV variants. The departure from positive C/D correlation in this patient is related to the existence of more than one genetically distant minority subpopulations before therapy ( Fig. 3 ). Collectively, the data suggest that for Patients 8–11, minority HBV subpopulations existing before treatment were direct ancestors of the lamivudine-resistant HBV variants, whereas the subpopulations that were dominant pre-therapy failed to become lamivudine-resistant. For Patients 6 and 7, however, the lamivudine-resistant variants mostly originated from the dominant pre-treatment subpopulations. Epistatic connectivity of lamivudine-resistance mutations The findings presented above indicate variation in the capacity of the intra-host HBV subpopulations to develop drug resistance, suggesting that fitness effects of drug-resistance mutations significantly depend on the genetic structure of HBV genome. Accordingly, the lamivudine-resistance phenotype is a complex trait encoded by the entire HBV genome rather than by single mutations and as such should be defined by epistatic connections among HBV genomic sites, with the primary and secondary lamivudine-resistance mutations being involved in these connections. To investigate this epistatic connectivity, we constructed a set of Bayesian networks (BNs) of polymorphic amino-acid sites in HBV proteins of pre-treatment and post-treatment viral populations from each patient ( Fig. 5 ). For Patients 8 and 9, BNs were constructed using only the pre-treatment subpopulations, which were genetically close to the resistant HBV variants. 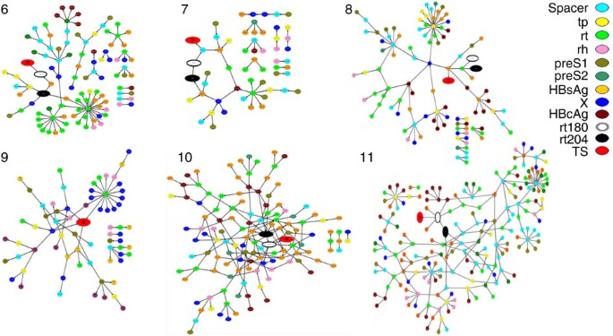Figure 5: BNs of intra-host HBV variants from Patients 6–11. Tp, spacer, rt and rh—terminal protein, spacer, RT and RNAse H domains of the HBV P protein; S1, S2 and hepatitis B surface antigen (HBsAg)—preS1, preS2 and S domains of the HBV S protein; X, the X protein; hepatitis B core antigen (HBcAg), the core protein; TS, sampling time, the variable describing sampling of HBV variants before or after lamivudine treatment. Figure 5: BNs of intra-host HBV variants from Patients 6–11. Tp, spacer, rt and rh—terminal protein, spacer, RT and RNAse H domains of the HBV P protein; S1, S2 and hepatitis B surface antigen (HBsAg)—preS1, preS2 and S domains of the HBV S protein; X, the X protein; hepatitis B core antigen (HBcAg), the core protein; TS, sampling time, the variable describing sampling of HBV variants before or after lamivudine treatment. Full size image In each patient, 45–100% of all polymorphic amino-acid sites were organized in a single network. In Patients 6 and 7, whose drug-resistant HBV variants mainly evolved from the major pre-treatment subpopulations, only 66 (58%) and 28 (45%) sites, respectively, were involved in BN. In Patients 8, 9, 10 and 11, whose drug-resistant HBV variants evolved from minority subpopulations, the number of sites in BN varied from 66 to 202 (76–100% of all polymorphic sites). HBV BN from Patients 6, 7, 8, 10 and 11 included rt204 and rt180, indicating that the state of these lamivudine-resistance sites depends on other sites in the HBV genome. The lamivudine-resistance sites were found to be significantly interrelated to each other and to several sites from the HBV C, S, X and P proteins ( P <0.0001; Fig. 5 ). HBV resistance to lamivudine is considered to be primarily associated with point mutations, such as rtM204I/V and rtA181V/T (ref. 3 ). The data presented in this study indicate that, although essential, the mere presence of rtM204V/I is not sufficient for the development of the HBV lamivudine-resistance. For example, single HBV variants that carried the rtM204I substitution before therapy in Patients 6 and 9 were unsuccessful in establishing detectable intra-host HBV populations after treatment. For Patient 6, the lamivudine-resistant HBV population originated mainly from the pre-treatment majority variant. In Patient 9, the pre-treatment rtM204I-carrying variant belonged to genotype G but only recombinant A/G variants became established after treatment. The calculated high rate of mutations ranging from 10 −4 to 10 −5 mutations per site per year [11] , [12] coupled with the estimated daily production of HBV in excess of 10 11 –10 13 virions [13] , [14] theoretically can result in daily generation of all single substitutions at each site of the HBV genome [5] or even all possible double substitutions [14] . Thus, the lamivudine-resistance substitutions may readily emerge during the course of HBV infection and be present in the intra-host HBV population in patients who have not been exposed to treatment. Indeed, these substitutions were recently detected by ultra-deep sequencing of HBV variants from treatment-naïve and lamivudine-treated patients [15] . The observations of two large HBV subpopulations (both developing lamivudine resistance) in Patient 1, the lamivudine-resistant minority subpopulations in Patients 5, 6 and 11 and more than one type of lamivudine-resistance mutations in Patients 2, 3 and 10 strongly support this supposition of frequent presentation of lamivudine-resistance substitutions. In each case, the lamivudine-resistance substitutions have been independently acquired by more than one HBV variant, indicating recurrent, convergent evolution toward lamivudine resistance in patients who developed breakthrough infection. The observed homoplasy and convergence rooted in the high rate of mutations are not compatible with the commonly assumed origination of the intra-host drug-resistant viral populations from a single viral clone. The development of lamivudine resistance in the patients studied here cannot be explained by the random presentation of point mutations. The emergence of these mutations is not a limiting factor in the development of drug resistance. Rather, our data indicate that the genetic structure of the HBV genome is critical in selecting variants capable of taking advantage of these mutations under the selection pressure of antiviral therapy. The differential capacity of the intra-host HBV subpopulations to lamivudine resistance observed in Patients 8, 9, 10 and 11 suggests that the fitness effects of lamivudine-resistance mutations varied depending on the genetic composition of the viral genome. This supposition is strongly supported by analysis of BNs connecting polymorphic amino-acid sites from HBV proteins in Patients 6–8, 10 and 11. These networks showed that the states of rt204 and rt180 are strongly associated with the states of many other sites from all HBV proteins, thereby highlighting the role of epistatic connectivity and coevolution among sites across the entire HBV genome in the development of drug resistance [6] . Finally, findings from this study suggest that differential predisposition to drug-resistance for HBV variants is a more realistic framework for understanding disparity in the development of drug resistance among patients than the fortuitous emergence of resistance mutations. This predisposition can be assessed and used to predict response to treatment. As predisposition to resistance is defined by the entire genome rather than by a single independent mutation, it cannot revert upon cessation of treatment. Lamivudine is widely used in treating patients with HBV mono-infection particularly in resource-limited countries and is an important component of anti-retroviral therapy for patients co-infected with HBV and human immunodeficiency virus. Thus, the widespread use of lamivudine favors selection of HBV variants with genetic composition that is predisposed to resistance to this drug, potentially leading to a genetic shift in the HBV population toward the increased resistance. Although lamivudine is no longer a first-line drug in developed countries, the concept as proposed here should be applicable to other antiviral drugs. Furthermore, HBV variants resistant to lamivudine are also resistant to telbivudine and less susceptible to entecavir [16] , [17] , indicating that selection for lamivudine resistance may result in increased likelihood of cross-resistance to other drugs. Therefore, our findings may have implications for improving the efficacy of antiviral therapy against HBV infection. HBV whole-genome quasispecies analysis Full-length HBV genome was amplified by two rounds of PCR [11] . Briefly, the first round of PCR was conducted using the primer combination of HBV1823FLong and HBV1801RLong ( Table 2 ). The thermal profile for the first-round amplification was as follows: 94 °C for 3 min (hold), ten cycles of 94 °C for 20 s, 55–45 °C for 30 s with step-down of 1 °C per cycle and 68 °C for 4 min; 35 cycles of 94 °C for 20 s, 45 °C for 30 s, 68 °C for 4 min with increasing elongation time for 10 s per cycle to 7 min 20 s and the final elongation at 68 °C for 10 min. The first-round PCR was performed on the GeneAmp PCR system 9,700 (Applied Biosystems, Foster City, CA, USA) using the Expand High-Fidelity PCR test kit. The second-round PCR was conducted using six sets of primers (set 1: HBV1847FS and HBV2394RS, set 2: HBV2298FS and HBV2933RS, set 3: HBV2821FS and HBV0272RS, set 4: HBV0179FS and HBV0704RS, set 5: HBV0599FS and HBV1286RS and set 6: HBV1175FS and HBV1788RS) for amplification of six overlapping fragments ( Table 2 ) under the following cycling conditions: 95 °C for 10 min (hold), 40 cycles of 95 °C for 10 s, 45 °C for 10 s and 72 °C for 32 s. The nested amplification was performed by using the Mx3005P SYBR Green Real-Time PCR System (Stratagene, La Jolla, CA, USA). The derivative melting curves were obtained using the instrument data analysis software. Table 2 PCR primers. Full size table End-point limiting-dilution-PCR was performed using serially diluted DNA [18] . Dilution, at which 20–30% of PCR repeats were found positive, was considered as the endpoint. Nested PCR of the 441-bp fragment of the S gene (primer set 4) was used to establish this condition. All six sets of PCR fragments were amplified using the same end-point dilution. Clone selection, serial dilution and reagent dispensing were performed using the Biomek 3,000 robotic station (Beckman-Coulter, Brea, CA, USA). Approximately 30–40 whole-genome clones were amplified from each sample. The number of clones varied depending on viral titre of samples. Genetic analysis Multiple sequences alignment was performed using programmes in Accelrys GCG, Version 11.0. (Genetic Computer Group, Accelrys Inc., San Diego, CA, USA). The extent of HBV genetic diversity for each patient was measured as the average Sn over all genomic positions. Sn of each position was measured as S =−Σ( p i ln p i ), where p i is the frequency of each nucleotide. The normalized entropy Sn= S /ln N was calculated to take into consideration the total number of sequences (N) obtained in each patient. To test whether the HBV genetic diversity was significantly changed between the pre- and post-treatment in each patient, we performed a paired samples t -test for all HBV genomic positions. AMOVA was used to identify positions with significant changes of nucleotide frequency between HBV variants found before and after lamivudine treatment. Estimates of st were used to analyse the genetic structure of HBV population by taking into consideration differences in frequency and composition of sequence variants. AMOVA was calculated using the program ARLEQUIN [19] ; significance levels of the genetic variance components were estimated using a permutation test ( n =10,000). Phylogenetic analysis The program ModelTest [20] was used to establish the best model of nucleotide substitution for the HBV data. The GTR model was chosen to create maximum likelihood trees [21] using the program HyPHY [22] . The initial tree was created using the neighbour-joining approach [23] , a search in the tree space was performed using nearest neighbor interchange of branches on the tree until no further likelihood score improvements could be made. Maximum likelihood distance matrix The program HyPHY [22] was used to create a maximum likelihood distance matrix [21] among HBV sequences. This distance matrix was used to create a scatterplot, where each pre-lamivudine sequence was plotted according to its value in two dimensions: the average distance to all other pre- or post-treatment sequences. Bayesian network Relationships among HBV protein sites from pre- and post-treatment populations were examined using probabilistic graphical models in the form of BNs [24] . For each patient, the aligned sequences were associated with the sampling time; namely, pre- or post-treatment. States of polymorphic sites and sequence sampling time-point constituted the entire set of viral features. Sequence deletions in HBV variants were also encoded as a feature and represented as a node in BN. Learning of the BN structure was based on the Greedy Thick Thinning method [25] , where the structure was constrained so that any given node in BN could have no greater than three parents. Estimation of the conditional probabilities was performed using the K2 priors of each feature [26] . In addition, relationship analysis of the HBV BN was performed to infer significance/strength of relationships between the features. The strength of the probabilistic relations between variables that it represents in the global probability law was measured by computing the Kullback–Leibler (KL) divergence [27] between the joint probability distribution of a relation with and without the arc. This is a measure of dependence between variables. The P -values represent the independence probabilities of the G-KL–test computed on the BN for each relationship, where G-KL is the independence G test of KL divergence of the relationship in the network. This analysis was done using the BayesiaLab (v4.6) software package (Bayesia SAS, Laval, France). Nucleotide sequence accession numbers The whole-genome sequences produced in this study have been deposited in the National Center for Biotechnology Information GenBank database under accession numbers JQ707299 to JQ707774 . Ethics statement Serum specimens of all patients were acquired with written informed consent, and the study involving human participants was approved by the Institutional Review Board of Centers for Disease Control and Prevention. How to cite this article: Thai, H. et al . Convergence and coevolution of Hepatitis B virus drug resistance. Nat. Commun. 3:789 doi: 10.1038/ncomms1794 (2012).